Loss of wild-type p53 promotes mutant p53-driven metastasis through acquisition of survival and tumor-initiating properties Missense-type mutant p53 plays a tumor-promoting role through gain-of-function (GOF) mechanism. In addition, the loss of wild-type TP53 through loss of heterozygosity (LOH) is widely found in cancer cells. However, malignant progression induced by cooperation of TP53 GOF mutation and LOH remains poorly understood. Here, we show that mouse intestinal tumors carrying Trp53 GOF mutation with LOH (AKTP M/LOH ) are enriched in metastatic lesions when heterozygous Trp53 mutant cells (AKTP +/M ) are transplanted. We show that Trp53 LOH is required for dormant cell survival and clonal expansion of cancer cells. Moreover, AKTP M/LOH cells show an increased in vivo tumor-initiating ability compared with AKTP Null and AKTP +/M cells. RNAseq analyses reveal that inflammatory and growth factor/MAPK pathways are specifically activated in AKTP M/LOH cells, while the stem cell signature is upregulated in both AKTP M/LOH and AKTP Null cells. These results indicate that TP53 / Trp53 LOH promotes TP53 / Trp53 GOF mutation-driven metastasis through the activation of distinct pathway combination. Colorectal cancer (CRC) is a leading cause of cancer-related death around the world [1] , [2] . The most frequently mutated gene in the pan-cancer cohort is TP53 [3] , and its mutations in CRC are detected in about 55–60% of cases [4] , [5] . During the malignant progression of CRC, TP53 mutations occur near the transition from benign to malignant lesion [6] , and indeed, the mutation incidence was shown to be about 80% when metastasis-associated CRCs were examined [7] . These results suggest that TP53 mutations play a role in the promotion of malignant progression in CRC. Unlike other tumor suppressor genes, the majority of TP53 mutations are missense-type at hot spots, resulting in the expression of mutant p53 protein with a single amino acid substitution [8] , [9] . It has been shown that such mutant p53 plays an oncogenic role through a gain of function (GOF) mechanism. For example, mouse models expressing mutant p53 R172H and p53 R270H (mutation at codons 175 and 273 in humans) developed adenocarcinomas in the intestine and lung that were not found in Trp53 -disrupted p53 Null mice [10] , [11] . In addition, p53 R172H mice demonstrated metastasis of pancreatic cancer [12] , and we recently showed that the expression of p53 R270H induces the submucosal invasion of intestinal tumors in an Apc Δ716 mouse model [13] , [14] . Importantly, the ablation of mutant p53 expression in cancer cells suppressed transplanted tumor growth in vivo and extended the animal survival, indicating that tumor growth is dependent on the sustained expression of mutant p53 [15] . Mechanically, it has been shown that the expression of mutant p53 results in expansion of mammary epithelial stem cells [16] and that mutant p53 induces stem cell gene signatures in CRC as well as mesenchymal stem cell-derived tumors [17] , [18] . These results suggest that mutant p53 promotes the late stage of tumorigenesis, possibly through the acquisition of an invasive ability and stem cell characteristics. Several molecular mechanisms underlying the involvement of mutant p53 in malignant progression have been reported, including constitutive activation of integrin and epidermal growth factor receptor (EGFR) signaling and the activation of TGF-β-dependent migration and PDGF receptor signaling [19] , [20] , [21] . In addition, it was recently shown that mutant p53 induces global transcriptional shift by epigenetic switching through interaction with the chromatin remodeling complex or the modification of histone methylation and acetylation [22] , [23] . In addition to these acquired oncogenic functions of mutant p53, the loss of wild-type p53 through the loss of heterozygosity (LOH) is found in >93% of human cancers [24] . This loss also plays an important role in malignant progression. We and other groups have shown that Trp53 LOH is important for the stabilization and nuclear accumulation of the mutant p53 [13] , [14] , [25] . However, the in vivo mechanism underlying the combination of the expression of GOF mutant p53 and loss of wild-type p53 by LOH for malignant progression is poorly understood. We previously generated an intestinal tumor metastasis model by splenic transplantation of mouse intestinal tumor-derived organoids, termed AKTP +/M cells, that carry Apc Δ716 , Kras +/G12D , Tgfbr2 -/- and Trp53 +/R270H mutations simultaneously [26] . These four-driver genes are included among the frequently mutated genes in human CRC [3] , [4] and are well-characterized as genes responsible for the promotion of CRC multistep tumorigenesis [27] . In the present study, we investigate the role of the loss of wild-type Trp53 by LOH in the liver metastasis of AKTP +/M cells carrying a heterozygous Trp53 GOF mutation. We report that Trp53 LOH in combination with the expression of GOF mutant p53 is required for the survival of disseminated cancer cells and subsequent clonal expansion, which leads to metastasis development. We also show that inflammatory and MAPK pathways in addition to the stem cell pathway are activated in AKTP M/LOH cells. These results provide a mechanism involving GOF mutant p53 together with loss of wild-type p53 for acceleration of metastasis, findings that will contribute to the future development of therapeutic strategies against CRC metastasis. Enrichment of Trp53 LOH cells in liver metastasis tumors We previously generated intestinal tumor-derived organoid cells (AKTP +/M cells) from compound mutant mice, in which genetic alterations were simultaneously introduced to four colon cancer driver genes: Apc , Kras , Tgfbr2 , and Trp53 [26] . The genotype of Trp53 in AKTP +/M cells is heterozygous (+/R270H), which is one of Trp53 GOF mutations [8] , [9] . When AKTP +/M cells were transplanted to the spleen of immunodeficient mice (Fig. 1a ), multiple metastatic tumors developed in the liver with 100% incidence, which is consistent with the previous report [26] (Fig. 1b ). Histologically, the metastasized tumors in the liver showed an advanced malignant phenotype compared with the primary tumors in the spleen, including an epithelial-mesenchymal transition (EMT)-like structure and the generation of fibrotic microenvironment with α-smooth muscle actin (SMA)-positive myofibroblasts and the deposition of collagen fibers in the stroma (Fig. 1c ). These results suggest that transplanted tumor cells acquired malignant characteristics during the metastasis process. Fig. 1: Enrichment of Trp53 LOH cells in liver metastasized tumor cells. a Strategy for liver metastasis development in NSG mice. b Representative photographs of the spleen and liver at 4 weeks after transplantation, and histology sections of dashed lines (H&E). Bars, 10 mm. c Representative histology of liver metastases (top) and primary spleen tumors (bottom). H&E, immunohistochemistry for p53, double-fluorescence immunostaining for α-smooth muscle actin (αSMA) and E-cadherin (Ecad) and Masson Trichrome staining (left to right). The insets show enlarged images. Bars, 100 µm. d Representative results of genomic polymerase chain reaction (PCR) for Trp53 in AKTP +/M cells (left) and spleen and liver tumors (right top). Each lane indicates the tumor cells collected from independent tumors in the spleen and liver. Mut Trp53 and WT Trp53 indicate mutant Trp53 R270H and wild-type Trp53 , respectively. The AKTP +/M organoid DNA was used as control. The band intensities (WT Trp53 /Mut Trp53 ) were quantified using ImageJ, and relative band intensities of each sample in spleen (blue bars) and liver (magenta bars) to that of control (closed bar) are indicated as bar graph ( n = 1 for each bar corresponding to each band) (bottom). LOH, loss of heterozygosity. e The mean relative band intensities in spleen tumors (blue) and liver tumors (magenta) indicated in ( d ) are shown. Note that the level of the mean band intensity was significantly decreased in LOH tumors in the liver. f The ratio of tumor cells with p53 nuclear-only accumulation in the spleen and liver tumors are indicated by different colors, blue, 0–20%; purple, 20–40%: yellow, 40–60%, orange, 60–80%, and red, 80–100%. The nuclear accumulation of p53 was examined in 100 tumor glands (>20 cells/gland) for 6 microscopic fields. g The mean ratios of tumor glands containing nuclear-only p53 cells at >80% in spleen tumors (blue) and liver tumors (magenta) are shown. The data in e , g are presented as mean ± s.d. Two-sided unpaired t -test was used for statistical analysis. p values are provided; ns, not significant. In e , n = 8 (spleen tumors) and n = 4 (non-LOH or LOH liver tumors) biologically independent samples. In g , n = 6 biologically independent samples. Source data are provided as a Source data file. Full size image In the human CRC cells carrying TP53 mutations, loss of wild-type TP53 by LOH is frequently found [4] , [24] , suggesting that the combination of fa TP53 GOF mutation and the subsequent loss of wild-type TP53 is important for the acquisition of a malignant phenotype. To determine whether or not the wild-type Trp53 gene was lost in the metastasized AKTP cells, we collected tumor cells from paraffin-embedded sections of the spleen and liver tissues through laser microdissection (Supplementary Fig. 1 ) and performed Trp53 allele-specific genomic polymerase chain reaction (PCR). We confirmed that the PCR system detected both mutant and wild-type Trp53 simultaneously (Fig. 1d left). Of note, the relative band intensities of the wild-type Trp53 were decreased significantly in 4 out of 8 liver metastasized tumor samples compared with that in the parental organoid cells, while those in all spleen tumor samples were at a similar level to the control organoid, indicating that the tumor cells that carried GOF mutant Trp53 and lost wild-type Trp53 (hereafter AKTP M/LOH cells) were enriched in the metastatic tumors. (Fig. 1d right, e). It has been shown that loss of wild-type Trp53 enhances the stabilization and nuclear accumulation of mutant p53 [13] , [25] . Notably, the ratios of p53 nuclear accumulation without cytoplasmic distribution (nuclear-only accumulation) were higher in the liver metastasized tumor cells than in the primary spleen tumor cells (Fig. 1c, f ). We further confirmed that the number of tumor glands with increased p53-nuc only cells (>80%) was significantly higher in the liver tumors than in the spleen tumors (Fig. 1g ). Trp53 LOH for clonal expansion of dissociated single cells During the metastasis process, disseminated tumor cells are exposed to cellular stress, such as a dormant state and clonal proliferation [28] . To examine whether such stresses constitute selection pressure for the enrichment of AKTP M/LOH cells in the metastatic foci, we performed in vitro subcloning experiments (Fig. 2a ). We confirmed that wild-type Trp53 remained in AKTP +/M cells when cells were cultured in Matrigel with serial passages by mechanical dissociation with pipetting, with cells remaining as tumor glands rather than dissociating into single cells (Fig. 2a, b ). In contrast, when AKTP +/M cells were enzymatically dissociated by trypsin to single cells and subjected to subcloning on the culture dish, all subclones derived from the surviving cells showed loss of wild-type Trp53 , indicating that Trp53 LOH is required for the survival and clonal expansion of single dissociated cells (Fig. 2c ). In addition, single-cell subcloning of ATP +/M and AKP +/M cells that carried the heterozygous Trp53 GOF mutation in addition to Apc Tgfbr2 and Apc Kras compound mutations, respectively, also lost wild-type Trp53 in all surviving and expanded cell clones at 100% frequency (Fig. 2c ). We confirmed that the rate of p53 nuclear-only accumulation was significantly higher in AKTP M/LOH organoid cells than in AKTP +/M cells (48.0% and 6.8%, respectively). In contrast, the majority of AKTP +/M cells showed nuclear/cytoplasmic (73.0%) or cytoplasmic-only p53 distribution (11.6%), which were rarely found in AKTP M/LOH cells (Fig. 2d, e ). Fig. 2: Selection of Trp53 LOH cells in the subcloned intestinal tumor cells. a Schematic drawing of the Trp53 LOH analysis. The organoids were mechanically dissociated by pipetting and passaged into Matrigel or were enzymatically dissociated to single cells and subcloned on culture dishes. b Representative genomic PCR results of Trp53 of AKTP +/M organoids maintained in Matrigel with mechanical passage (p, passage number). Mut Trp53 and WT Trp53 indicate mutant Trp53 R270H and wild-type Trp53 , respectively. Molecular weight marker for Trp53 allele-specific PCR is shown in Fig. 1d . The experiments shown in ( b ) were repeated three times with similar results, and the representative results are shown. c Genomic PCR results of Trp53 of independent subclones from AKTP +/M , ATP +/M , AKP +/M , and AKTFP +/M organoids. Genomic DNAs of AKTP +/+ , AKTP M/M , and AKTP +/M cells were used as controls. The numbers of Trp53 LOH subclones per total subclones are indicated in parentheses. The band intensities (WT Trp53 /Mut Trp53 ) of AKTPF subclones were quantified using ImageJ, and relative band intensities of each subclone (blue bars) to that of control (closed bar) are indicated as bar graph ( n = 1 for each bar corresponding to each band) (bottom). ND, not detected. d Representative confocal images of AKTP M/LOH (left) and AKTP +/M (right) organoids immunostained for p53 and E-cadherin (Ecad) with DAPI nuclear staining are shown. The insets indicate enlarged images. Bars, 100 µm. e The percentages of p53 subcellular localization with nuclear-only (Nuc), mixed nuclear and cytoplasmic (Nuc/Cyt), and cytoplasmic-only (Cyt) in the AKTP +/M (blue) and AKTP M/LOH (magenta) organoid cells are shown. The total numbers of examined cells/organoids are indicated. f The ratios of organoid development from single AKTP +/M cells (closed bar) and AKTP M/LOH cells (red bars) in type I collagen gel (left) and Matrigel (right) are shown. The numbers of developed organoids and seeded cells are provided. g The results of soft agar colony formation assay. The number of colonies and seeded cells are provided. The data in e , f are presented as mean ± s.d., n = 12 ( e ) and n = 3 ( f ) biologically independent samples. p values are provided; ND, not detected. Two-sided unpaired t -test was used to calculate statistical difference. Source data are provided as a Source data file. Full size image We next examined whether or not Trp53 LOH is required for the survival and clonal expansion in three-dimensional (3D) culture conditions. Consistent with two-dimensional (2D) culture experiments, trypsin-dissociated single AKTP M/LOH cells but not AKTP +/M cells formed organoids in collagen gel (Fig. 2f left). Although a small number of AKTP +/M cells survived and formed organoids in Matrigel, the organoid formation efficiency was significantly higher in AKTP M/LOH cells (Fig. 2f right). It is possible that signaling from the extracellular matrix (ECM) in Matrigel enhances the dissociated cell survival. These results, taken together, indicate that Trp53 LOH is important for the dormant cell survival and clonal proliferation of cancer cells, possibly through the increased nuclear accumulation of mutant p53. In contrast, neither AKTP M/LOH and AKTP +/M cells developed colonies in soft agar (Fig. 2g ), indicating that AKTP M/LOH cells have not yet acquired the ability to achieve anchorage-independent growth and thus may require signaling from the extracellular matrix (ECM) for clonal expansion. Interestingly, the efficiency of the Trp53 LOH cell enrichment through the subcloning decreased to 40% when the Fbxw7 gene was disrupted in AKTP +/M cells (namely AKTFP +/M cells) (Fig. 2c ). Of note, the genetic alterations in TP53 and FBXW7 in human CRC tend to be mutually exclusive, although the difference was not found to be significant (Supplementary Fig. 2 ). Accordingly, Trp53 LOH may not be essential for metastasis when the FBXW7 function is suppressed, although further investigations are needed. Mechanisms underlying Trp53 LOH in AKTP +/M cells We next confirmed the loss of wild-type Trp53 in AKTP M/LOH cells by direct sequencing, while both wild-type and mutant Trp53 were found in AKTP +/M cells (Fig. 3a ). CMT93 mouse colon cancer cells were used for the Trp53 wild-type cell control. To further examine the LOH mechanism in AKTP +/M cells, comparative genomic hybridization (CGH) analyses were performed for three independent AKTP M/LOH lines: 1C9, 2A6, and 3F9 (Fig. 3b ). We confirmed the euploidy status of parental AKTP +/M cells that were maintained in Matrigel by mechanical passages. Fig. 3: Mechanism underlying Trp53 LOH in AKTP +/M cells. a Direct sequencing of genomic DNA fragments including codon 270 (under line) of Trp53 in CMT93 cells, AKTP +/M , and AKTP M/LOH cells. WT, wild-type Trp53 ; and MT, mutant Trp53 (R270H). b A whole-genome CGH analysis of the indicated AKTP M/LOH subclones (1C9, 2A6, and 3F9) and parental AKTP +/M cells. Chr indicates chromosome number. c TaqMan SNP genotyping results of AKTP M/LOH 2A6 cells (open diamonds with red line), AKTP M/LOH 1C9 cells (red diamonds with black line), AKTP M/LOH 3F9 cells (magenta diamonds), AKTP +/M cells (green squares), AKTP +/+ cells (blue squares), and no template control (NTC) (yellow triangles) are shown as a scatter plot. The Trp53 allelic discrimination data are shown as a scatter plot of Trp53 wild-type codon 270 (CGT) (HEX dye) versus Trp53 mutant codon R270H (CAT) (FAM dye). Note that two AKTP M/LOH subclones (2A6 and 1C9) carry two copies of mutant Trp53 R270H, while one AKTP M/LOH subclone 3F9 carries one copy or Trp53 R270H. Source data are provided as a Source data file. Full size image In contrast, common copy number variations were found in AKTP M/LOH lines, such as Chr4 loss in 1C9 and 3F9 cells, suggesting the advantages of these copy number variations for overcoming subcloning stress. Notably, a decrease in the copy number of Chr11 containing the Trp53 gene was detected in 3F9, indicating the hemizygous status of mutant Trp53 in this subclone (one Trp53 R270H copy left in cells). Consistently, real-time genomic PCR using wild-type and mutant Trp53 -specific primers revealed that 1C9 and 2A6 cells contained two copies of the mutant Trp53 gene, namely copy-number-neutral LOH (AKTP M/M cells), while 3F9 cells carried a single copy of the GOF mutant Trp53 (Fig. 3c ). Notably, the protein levels of mutant p53 were similar in all three subclones (Supplementary Fig. 3 ). These results suggest that the copy number of the mutant p53 is not relevant for the survival and clonal expansion ability of cancer cells. For further analyses in this study, we used AKTP M/M cells as AKTP M/LOH cells. Protection from anoikis by Trp53 GOF mutation with LOH It has been shown that the disruption of cell-cell or cell-ECM contact causes intestinal epithelial cell death, known as anoikis [29] . p53 plays a role in the stress response through the induction of cell cycle arrest and apoptosis [30] , so the loss of wild-type p53 helps protect the dissociated single cells from anoikis at least in part. We, therefore, examined the cellular response to anoikis of AKTP M/LOH cells. For this experiment, we additionally constructed AKTP Null cells, in which both alleles of Trp53 in AKTP +/+ cells had been disrupted by the CRISPR/Cas9 system (Supplementary Fig. 4 ). AKTP Null cells developed cystic organoids in Matrigel, which were similar to AKTP +/+ and AKTP +/M organoids (Fig. 4a ). However, AKTP M/LOH formed complexed glandular structures, indicating that AKTP M/LOH cells acquired distinct characteristics from AKTP +/M and AKTP Null cells. Fig. 4: Increased survival of dissociated tumor cells by Trp53 GOF mutation with LOH. a Representative photographs of four AKTP organoid lines with different Trp53 genotypes (AKTP +/+ , AKTP +/M , AKTP Null , and AKTP M/LOH ). Bars, 500 µm. Note that AKTP M/LOH cells formed a complex glandular structure, while other organoids showed a round cystic structure. The images are representative of six independent cultures. b A flow cytometry analysis for cleaved caspase 3 (Casp3) of trypsin-dissociated cells of the four different Trp53 genotypes. Gating strategy is shown in Supplementary Fig. 5 . The apoptosis rate is indicated in each graph. c Cloning efficiencies examined by limiting dilution of trypsin-dissociated single cells in 96-well plates are shown as a bar graph. The numbers of 96-well plates used for each genotype analysis are indicated in parentheses. Cloning efficiency was calculated in each 96-well plate, and the mean cloning efficiency was calculated ( n = 6–9 biologically independent samples). Gray-line bar, AKTP Null cells; red-line bar, AKTP M/LOH cells; and ND, not detected. d , e The results of a cell proliferation assay of trypsin-dissociated single AKTP cells (500 cells/well) ( n = 3 biologically independent samples) ( d ) and mechanically dissociated AKTP cell clumps (~30 clumps containing 1–2 × 10 3 cells/Matrigel) ( n = 3 biologically independent samples) ( e ). Red lines with triangles, AKTP M/LOH cells; blue lines with circles, AKTP +/M cells; gray lines with triangles, AKTP Null cells; and black lines with squares, AKTP +/+ cells. The relative cell growth compared to the day 0 level is indicated. Data are presented as mean ± s.d. The data in c were analyzed by two-sided unpaired t -test, p values are provided; ND, not detected. The data in d , e were analyzed by ANOVA test, * p < 0.0001; ns, not significant. Data in d were also analyzed by Tukey test, p values at day 4 are provided. Source data are provided as a Source data file. Full size image Flow cytometry analyses showed that the rate of apoptosis of AKTP +/+ and AKTP +/M cells after trypsin-dissociation was similar (21.5% and 22.4%, respectively), indicating that the heterozygous Trp53 GOF mutation is not sufficient for protection from anoikis (Fig. 4b , Supplementary Fig. 5 ). As expected, the apoptosis rate of the trypsin-dissociated AKTP Null cells decreased significantly to 8.7%. Importantly, however, the apoptosis ratio was further suppressed to 1.0% in AKTP M/LOH cells, indicating that the combination of the Trp53 GOF mutation with LOH protects tumor cells from anoikis more efficiently than the biallelic loss of wild-type Trp53 . Consistently, AKTP M/LOH cells showed greater cloning efficiency than AKTP Null cells when a trypsin-dissociated single cell was seeded into each well of a 96-well plate (Fig. 4c ). AKTP +/+ and AKTP +/M cells failed to form colonies after single-cell dissociation in this assay. Similarly, the number of proliferated cells was significantly higher in AKTP M/LOH cells followed by AKTP Null cells compared with that in AKTP +/+ and AKTP +/M cells when 5 × 10 2 single-dissociated cells were seeded into each well of a 96-well plate (Fig. 4d ). In contrast, when the mechanically dissociated cells were cultured in Matrigel after passage, the survival and growth rates of tumor cells were relatively unchanged among the all Trp53 genotypes, regardless of the Trp53 genotypes (Fig. 4e ). These results, taken together, indicate that Trp53 LOH is not required for the survival and proliferation of tumor cells if cell-cell contacts are maintained as tumor glands. Tumor-initiation by Trp53 GOF mutation with LOH The acquisition of dormant cell survival and cloning expansion properties may be associated with the tumor-initiation capability. We, therefore, examined the in vivo tumor formation from a small number of AKTP cells with each Trp53 genotype by subcutaneous (s.c.) transplantation of 1 × 10 2 trypsin-dissociated cells per site in NSG mice (Fig. 5a ). AKTP +/M and AKTP Null cells developed 5 and 7 tumors, respectively, when injected at 14 sites (35.7 and 50%, respectively), while AKTP +/+ cells did not form any tumors (Fig. 5b, c ). Thus, either a heterozygous Trp53 mutation or the loss of the wild-type p53 function contributes to an increased tumor-initiation ability. Notably, AKTP M/LOH cells induced tumor development in 12 out of 14 injected sites (85.7% incidence), indicating that the combination of a Trp53 GOF mutation with LOH further accelerates tumor initiation from single cells. However, when the respective Trp53 genotype AKTP cells were mechanically dissociated (not to single cells) and transplanted at 5 × 10 3 cells per site, AKTP +/M , AKTP Null , and AKTP M/LOH cells induced tumor development at 11–12 of 15 injection sites (73.3–80%) (Fig. 5d, e ). These results suggest that the combination of a Trp53 GOF mutation with LOH is important for the development of tumor foci when a small number of single cells are disseminated. Fig. 5: Enhanced tumor-initiating ability by Trp53 GOF mutation with LOH. a Strategy of subcutaneous (s.c.) tumor development in NSG mice. b The s.c. tumor size changes in each site injected with 1 × 10 2 trypsin-dissociated cells of the indicated genotypes are shown as line graphs. The total number of injected sites ( n = 14) is indicated in each graph. Each line with closed or open circles, squares, diamonds, or triangles indicates the kinetic tumor size development of an individual tumor. c The total number of developed tumors ( y -axis) at the 14 injected sites is shown by red bars. Blue bars indicate number of sites where tumors did not develop. The ratio (%) of tumor development is indicated inside each bar. d The s.c. tumor size changes in each site injected with 5 × 10 3 mechanically dissociated cells of the indicated genotypes are shown as line graphs. The total number of injected sites ( n = 15) is indicated in each graph. Each line with closed or open circles, squares, diamonds, or triangles indicates the kinetic tumor size development of an individual tumor. e The total number of developed tumors ( y -axis) at the 15 injected sites is shown. The ratio (%) is indicated inside each bar. f Representative histology photographs of s.c. tumors that developed from 1 × 10 2 trypsin-dissociated cells. Cell genotypes are indicated in the left. H&E and immunohistochemistry for Ki67, p53, and double fluorescent immunohistochemistry for α-smooth muscle active (αSMA) (green)/E-cadherin (Ecad) (red) are shown. The insets show enlarged images. Bars, 200 µm. Source data are provided as a Source data file. Full size image Consistent with the liver metastasized tumors (Fig. 1c ), AKTP M/LOH s.c. tumors showed a poorly differentiated EMT-like histology with the generation of a fibrotic microenvironment characterized by increased αSMA-positive myofibroblasts, which was more advanced than in AKTP +/M and AKTP Null cell tumors (Fig. 5f ). However, no significant differences were noted in the Ki67-labeling indices among AKTP +/M , AKTP Null , and AKTP M/LOH tumor cells, indicating that the p53 status is important for dictating malignant cell characteristics, except for the proliferation rate (Supplementary Fig. 6 ). Metastasis-initiation by Trp53 GOF mutation with LOH We further examined the efficiency of metastatic foci development by the Trp53 genotype of AKTP cells using a small number of single cells by transplantation of 3 × 10 2 trypsin-dissociated cells to the spleen (Fig. 6a ). An intensive histological analysis of serial sectioning revealed small metastatic foci in the liver of three out of four mice that were transplanted with AKTP M/LOH cells (Fig. 6b, c ). We confirmed Wnt signaling activation by the Sox17 expression and proliferation of metastasized cells by Ki67 immunostaining (Fig. 6d ). In contrast, such metastatic foci were not found in the livers of mice transplanted with other Trp53 genotype AKTP cells (Fig. 6c ). These results support the hypothesis that the combination of a Trp53 GOF mutation and loss of wild-type Trp53 promotes metastasis development through the acquisition of survival and clonal expansion properties of disseminated dormant cells. Fig. 6: Enhanced metastasis-initiating ability of the Trp53 GOF/LOH tumor cells. a The strategy of metastasis tumor development in NSG mouse liver. A small number of trypsin-dissociated cells (3 × 10 2 cells) were injected into the spleen. The liver metastatic foci were examined by an intensive histological analysis. b Representative histology section of the whole liver lobe of a mouse injected with AKTP M/LOH cells (H&E) is shown. The arrowhead indicates a micrometastatic lesion consisting of AKTP M/LOH cells. Bar, 1 mm. The image is a representative of three independent mice that showed liver metastasis. c The numbers of metastatic tumor foci found in the liver in each mouse are shown with closed dots. Data are presented as mean ± s.d., n = 4 biologically independent animals. Wilcoxon’s nonparametric analysis was used to calculate statistical difference. p value vs. AKTP +/+ , AKTP +/M , and AKTP Null cells is provided; ND, not detected. d Representative histology of the serial sections of an AKTP M/LOH cell metastatic lesion (indicated lesion by dotted circle in b ); H&E and immunohistochemistry for Sox17 and Ki67 (left to right). Bars, 200 µm. The images are representative of three independent experiments. Source data are provided as a Source data file. Full size image Activated pathways by Trp53 GOF mutation with LOH We finally performed RNA sequencing of AKTP cells with the different Trp53 genotypes as well as adenoma cells carrying simple Apc mutation (A cells) as a control. By hierarchical clustering analysis, we extracted three sets of differentially expressed genes (DEGs): AKTP M/LOH and AKTP Null cell-specific, AKTP M/LOH cell-specific, and AKTP Null cell-specific DEGs (Fig. 7a ). An ingenuity pathway analysis (IPA) using DEG sets indicated that stem cell pathways were upregulated in both AKTP M/LOH and AKTP Null cells (Fig. 7b ). A StemChecker analysis using RNAseq data also indicated the acquisition of stem cell properties in both AKTP M/LOH and AKTP Null cells at a similar level (Supplementary Fig. 7 ). Importantly, a further IPA analysis indicated that growth factor/MAPK and inflammatory pathways were specifically activated in AKTP M/LOH cells but not in AKTP Null cells (Fig. 7c, d ). STRING database search indicated significant interaction among target molecules of these activated upstream regulators, suggesting that growth factor/MAPK and inflammatory pathways generate signaling network in AKTP M/LOH cells (Supplementary Fig. 8 ). Fig. 7: Activation of inflammatory and MAPK pathways by Trp53 GOF mutation with LOH. a A hierarchical clustering analysis of AKTP M/LOH and AKTP Null -specific DEGs (top), AKTP M/LOH -specific DEGs (middle) and AKTP Null -specific DEGs (bottom) are shown as fold changes of RPKM compared with the mean. Color scale represents the Z-score log2 intensity. For Trp53 genotypes, Wt, AKTP +/+ ; He, AKTP +/M ; Lo, AKTP M/LOH ; and Nu, AKTP Null . The color in the squares on the right of heatmap indicates genes that are upregulated (red) or downregulated (green) compared to A organoid. b – d The results of upstream regulator analyses by the Ingenuity Pathway Analysis software program using the AKTP M/LOH -specific DEGs (magenta bars), AKTP Null -specific DEGs (purple bars), and AKTP M/LOH & AKTP Null -specific DEGs (blue bars) mentioned in ( a ) are shown in bar graphs. Upstream regulators for the stem cell pathways with Z-scores > 2.0 in AKTP M/LOH & AKTP Null -specific DEGs ( b ), the growth factor/MAPK pathway with Z-scores > 2.0 ( c ) and the inflammatory pathway with Z scores > 3.0 in AKTP M/LOH -specific DEGs ( d ) are extracted and pathways with Z-scores > 1.5 are indicated as bars. e Cloning efficiencies of trypsin-dissociated AKTP M/LOH cells in the presence or absence of trametinib examined by limiting dilution in 96-well plates are shown ( n = 4 biologically independent samples). f The results of a cell proliferation assay of trypsin-dissociated single AKTP M/LOH cells (500 cells/well) in the presence or absence of trametinib (mean ± s.d.) ( n = 4 biologically independent samples). Data are presented as mean ± s.d. The data in e were analyzed by two-sided unpaired t -test, p value is provided; ND, not detected. The data in f were analyzed by ANOVA test, * p = 0.0994 at day 2, and ** p = 0.0012 at day 3. The data in f were also analyzed by Tukey test, p values at day 3 are provided. Source data are provided as a Source data file. Full size image We thus examined the role of the MAPK pathway in the acquisition of metastatic ability of AKTP M/LOH cells by treatment with the MEK inhibitor trametinib. Notably, trametinib treatment significantly suppressed the cloning efficiency of single-dissociated AKTP M/LOH cells (Fig. 7e ). Moreover, the proliferation of AKTP M/LOH cells after seeding 5 × 10 2 single-dissociated cells into a 96-well plate was significantly suppressed by treatment with trametinib (Fig. 7f ). Taken together, these results indicate that the loss of wild-type p53 causes the upregulation of the stem cell signature, while the cooperation of the mutant p53 expression and Trp53 LOH further activates the growth factor/MAPK and inflammatory pathway, which may promote metastasis through the acquisition of single cell survival and clonal expansion ability (Fig. 8 ). Fig. 8: A schematic illustration of the for TP53 / Trp53 mutation and metastasis. Loss of wild-type p53 increases stemness, while combination of p53 GOF mutation with LOH activates inflammatory and MAPK pathway. Corporation of these pathways may cause acquisition of single-cell survival and clonal expansion abilities, which promotes metastasis. Full size image A recent genome analysis indicated that major driver mutations, including TP53 , accumulate in the primary tumor cells at the early stage of tumorigenesis [31] , but the molecular mechanism underlying metastasis has not been genetically explained yet. The majority of TP53 GOF mutations are followed by loss of wild-type TP53 by LOH, and the possible mechanism underlying TP53 LOH for tumorigenesis was closely examined through cell line studies [32] . However, exactly when TP53 LOH is induced during tumorigenesis and what advantages it provides to cancer cells for malignant progression remain unclear. In the present study, we showed that cancer cells that lost wild-type Trp53 by LOH were selectively enriched in the metastatic foci when cancer cells carrying a heterozygous Trp53 mutation were transplanted in the primary site, indicating that the loss of wild-type Trp53 by LOH is required for metastasis. Furthermore, in the in vitro analyses, we showed that Trp53 LOH is not required for the survival or proliferation of cancer cells when they are maintained as tumor glands. However, Trp53 LOH is critical for the survival when cells are dissociated into single cells. These results indicate that Trp53 LOH is an important genetic alteration step for the survival of disseminated cells during metastasis. The next question is whether or not GOF mutant p53 is required for Trp53 LOH-associated metastasis. The loss of wild-type p53 causes the protection of dissociated tumor cells from apoptosis by the loss of p53’s functions against stress responses. However, the present results indicate that the survival rate of enzymatically dissociated cells is significantly higher in AKTP M/LOH cells than in AKTP Null cells. Furthermore, in vivo tumorigenesis from a small number of dissociated single cells is more efficient in AKTP M/LOH cells than in AKTP Null cells. These results indicate that GOF mutant p53 plays a role in the survival and proliferation of dormant cells in addition to the loss of wild-type p53; the combination of a GOF mutation and LOH is thus important for metastasis. However, it has been reported recently that the Trp53 null mutation and the combination of Trp53 R270H GOF/LOH mutations have similar effects on metastasis of intestinal tumors [33] . In this report, tumor phenotypes were examined using mice carrying Apc , Kras , and Trp53 (AKP) mutations, and metastasis was found in about 7–8% of both Trp53 null and Trp53 R270H/LOH mice, suggesting the need for additional genetic alterations in order to induce metastasis formation. It is, therefore, possible that the Trp53 null mutation is sufficient for inducing metastasis without a GOF mutation of Trp53 when specific genetic alterations other than AKTP mutations are accumulated. However, in line with the present results, it has been shown that a different type of GOF mutant Trp53 , R248Q, with loss of wild-type Trp53 induces an advanced malignant phenotype in an inflammation-associated colon cancer model when compared with Trp53 null mice [34] . Taken together, these present and previous findings strongly suggest that GOF mutant p53 proteins may be useful therapeutic targets, regardless of the mutation positions. An expression analysis showed that the stem cell signature is upregulated in both AKTP M/LOH and AKTP Null cells at similar levels, which may contribute to the tumor-initiating ability of cancer cells, although it is not sufficient for the induction of metastasis. However, the inflammation and growth factor/MAPK pathways are strongly activated in AKTP M/LOH but not in AKTP Null cells (Fig. 8 ). Inflammatory responses contribute to the generation of a fibrotic microenvironment in tumor tissue, and CRC with fibrotic stroma is classified as consensus molecular subtype (CMS)4, which is associated with a poor prognosis [28] , [35] . Consistently, we found a malignant histology of AKTP M/LOH cells in the metastatic tumors showing a rich fibrotic microenvironment (Figs. 1 c, 5f ). Furthermore, the activation of growth factor signaling, including that of EGF, PDGF, and VEGF, has also been reported in cancer cells carrying TP53 GOF mutations [19] , [21] , [23] . It is possible that signaling from a fibrotic microenvironment along with the cell-intrinsic activation of these growth factor pathways accelerate the acquisition of a tumor-initiating ability among CRC cells that express GOF mutant p53 and loss of wild-type p53. We extracted AKTP M/LOH -specific DEGs that are not upregulated or downregulated in AKTP +/M cells, indicating that the transcription of these genes requires the loss of wild-type p53 function. We previously found that wild-type p53 suppresses the nuclear accumulation of stabilized mutant p53 [13] , [14] . In the present study, we confirmed that the nuclear accumulation ratio of p53 was significantly higher in AKTP M/LOH cells than in AKTP +/M cells (Figs. 1f, g , and 2d, e ). Accordingly, it is possible that the loss of wild-type TP53 / Trp53 by LOH in the mutant TP53 / Trp53 heterozygous cells leads to the accumulation of mutant p53 in nuclei, which increases the expression of the mutant p53-specific gene set [13] . The loss of the tumor suppressor function of p53 is obviously important for malignant progression. However, the p53 nuclear accumulation may also be an important mechanism through which TP53 / Trp53 LOH promotes metastasis. In the present study, we found that AKTFP +/M cells, in which the Fbxw7 gene is disrupted, survived and expanded from dissociated single cells without the loss of wild-type Trp53 . Fbxw7 is a ubiquitin ligase that targets oncogenic proteins, including c-Myc [36] . It has been reported that mutant p53 contributes to tumorigenesis by allowing the overexpression of c-Myc through the downregulation of Fbxw7 [37] . Thus, the suppression of the Fbxw7 function causes the stabilization of c-Myc without a Trp53 mutation, which may contribute to the cell survival and proliferation. According to genome research results, certain populations of cancer cells retain intact TP53 [4] . Therefore, it is possible that Fbxw7 disruption induces the malignant progression of CRCs that carry intact TP53 . Using mouse intestinal tumor cells that carry quadruple driver mutations for Apc , Kras , Tgfbr2 , and Trp53 , we showed that cells remained sensitive to anoikis if their Trp53 status was heterozygous, and a loss of wild-type Trp53 by LOH is necessary for the cells to survive in a dormant state and proliferate toward metastasis. We further showed that the inflammation and MAPK pathways were activated by the combination of a Trp53 GOF mutation with LOH, which may contribute to the acquisition of a malignant phenotype among CRC cells. These results suggest that the inhibition of the mutant p53 function or suppression of TP53 LOH will be effective for preventing CRC metastasis. Tumor organoid cell lines We previously established AKTP +/M , ATP +/M , AKP +/M , AKF, and AKTFP +/M organoid cell lines from mouse intestinal tumors carrying mutations in the combinations of Apc Δ716 Kras +/G12D Tgfbr2 −/− Trp53 +/R270H , Apc Δ716 Tgfbr2 −/− Trp53 +/R270H , Apc Δ716 Kras +/G12D Trp53 +/R270H , Apc Δ716 Kras +/G12D Fbxw7 −/− and Apc Δ716 Kras +/G12D Tgfbr2 −/− Fbxw7 − / − Trp53 +/R270H , respectively [26] . These organoid cells carry heterozygous Trp53 R270H mutations. AKTP Null cells were generated by the disruption of Trp53 in AKT (AKTP +/+ ) cells. In brief, Trp53 CRISPR/Cas9 plasmid (Santa Cruz) was transfected to AKT cells by Lipofectamine LTX, and Trp53 disrupted cells were selected by the addition of 10 µM Nutlin-3 to the culture medium. These organoid cells were cultured in growth factor-reduced (GFR)-Matrigel (Corning) or culture dish with Advanced DMEM/F-12 medium (Gibco) supplemented with 10 mM HEPES, 2 mM Glutamax, 1×B27, 1×N2 (Invitrogen), 100 ng/ml murine Noggin (Peprotech) and 1 µM N-acethylcysteine (Sigma). For the passage of the organoids, organoid cells were recovered from Matrigel by a Cell Recovery Solution (Corning). They were then roughly broken up by pipetting (mechanical dissociation) using 1-ml tips, split and passaged into fresh Matrigel. For the enzymatic dissociation of organoids to single cells, the recovered organoids were treated with 0.25% trypsin at 37 °C for 5 min, and cells were then filtrated using a 35-µm mesh cell strainer (FALCON). The organoids were immunostained using antibodies for p53 (Leica Biosystems) at 1:200 and E-cadherin (R&D system) at 1:100, and Alexa Fluor 594- or Alexa Fluor 488-conjugated antibodies (Molecular Probes). The immunostained organoids were examined using confocal microscope, Leica TCS SP8 (Leica Microsystems), and the number of cells with p53 nuclear accumulation was scored and the ratio was calculated as nuclear p53 index. Mouse experiments Female NOD/Shi- scid Il2rg −/− (NSG) mice between 6 and 7 weeks of age were purchased (Charles River) for use in transplantation experiments. For the liver metastasis experiments, mechanically dissociated AKTP +/M organoid cells (1 × 10 5 cells/mouse) were injected into mouse spleen, and liver metastases were examined at 4 weeks after the injection ( n = 5). For s.c. tumor development, trypsin-dissociated organoid cells (1 × 10 2 cells/site) or mechanically dissociated organoid cells (5 × 10 3 cells/site) were injected s.c. (4–5 sites/mouse, and 4 mice each for different cell preparations and genotypes), and the tumor sizes (major diameter, mm) were measured every week until 12 weeks after injection. For in vivo tumor-initiation experiments, trypsin-dissociated organoid cells (3×10 2 cells/mouse) were injected into the spleen ( n = 4), and then the spleen was removed immediately after injection. At 8 weeks after the injection, all liver lobules were collected and processed for histology. Ten paraffin sections (80-µm intervals each) were prepared by microtome and examined. The metastasis frequency was calculated as the number of foci/1000 mm 2 . The mice were housed in a 12-h light/dark cycle at 23 °C ± 2 °C room temperature with relative humidity of 50 ± 20%, and given ad-libitum access to food and water for the duration of the study. Mice were housed in specific-pathogen-free (SPF) facility of Kanazawa University, Japan, and cared for in accordance with Fundamental Guidelines for Proper Conduct of Animal Experiment and Related Activities in Academic Research Institutions under the jurisdiction of the Ministry of Education, Culture, Sports, Science and Technology of Japan. All animal experiments were carried out according to the protocol approved by the Committee on Animal Experimentation of Kanazawa University, Japan. Histology and immunohistochemistry The spleen tumors, liver metastasis tumors, and s.c. tumors were fixated in 4% paraformaldehyde, paraffin-embedded, and sectioned at 4 - μm thickness. The sections were stained with H&E or Masson Trichrome. For immunohistochemistry, antibodies against αSMA (Sigma) at 1:800, E-cadherin (R&D Systems) at 1:100, p53 (CM5) (Leica Biosystems) at 1:200, Ki67 (Abcam) at 1:1000 and Sox17 (R&D Systems) at 1:100 were used as the primary antibody. Staining signals were visualized using the Vectastain Elite Kit (Vector Laboratories). For fluorescent immunohistochemistry, Alexa Fluor 594- or Alexa Fluor 488-conjugated antibodies (Molecular Probes) were used as the secondary antibody. The numbers of p53 nuclear-accumulated cells in the liver metastasis foci were scored in 5 microscopic fields, and the ratio was calculated as the mean number of positive cells per tumor gland. Proliferation analysis The number of Ki67 positive tumor cells and total tumor cells were counted in 5 independent microscopic fields (×200) for 3 independent tumors ( n = 15 for each genotype), and Ki67 labeling indices were calculated. Immunoblotting Organoid cells were lysed in lysis buffer, and protein samples were separated in 10% SDS-polyacrylamide gel. Antibodies for p53 (Cell Signaling Technology) was used. An anti-β-actin antibody was used as the internal control. The ECL detection system (GE Healthcare) was used to detect the signals. Band intensities were measured using ImageJ application. Trp53 LOH analyses To examine the Trp53 LOH, tumor cells were isolated from eight spleen tumors and eight liver tumors developed in six mice using LMD7000 laser microdissection (Leica Microsystems), and genomic DNA was purified using a NucleoSpin Tissue XS (Macherey-Nagel). Organoid cell-derived genomic DNA was used as a control. To detect the wild-type Trp53 and mutant Trp53 R270H , genomic DNA was amplified by PCR using a primer set for Trp53 (p53F1 and p53R1). Band intensities of the mutant Trp53 -specific band (330 bp) and wild-type Trp53 -specific band (290 bp) were measured using ImageJ, and the WT/Mut Trp53 ratio was calculated. Cell culture experiments For single-cell subcloning experiments, trypsin-dissociated single cells were plated on a collagen-coated dish or 96-well plates (1 cell/well) and cultured in advanced DMEM/F-12 medium supplemented with inhibitors for ROCK, 10 µM Y-27632 (Wako), GSK-3, 5 µM CHIR99021 (R&D) and TGF-β, 5 µM A8301 (Sigma). Genomic DNA was extracted from the subclones ( n = 5–17 for each genotype), and genomic PCR for Trp53 was performed to examine the LOH status. The cloning efficiency was examined by scoring the number of wells containing proliferated cells in the 96-well plates and calculating the ratios. For the organoid formation assay, 2.5 × 10 2 trypsin-dissociated single cells were cultured in 500 µl of collagen type I gel (Nitta gelatin), or 30 cell clumps including 1–2 × 10 2 cells were cultured in 30 µl of GFR-Matrigel. The numbers of developed organoids were counted at 14 days. For cell proliferation experiments, trypsin-dissociated single cells were plated in 96-well plates (5 × 10 2 cells/well), or 1 × 10 3 cells were cultured in 20 µl of GFR-Matrigel. The cell growth was examined by a CellTiter-Glo Luminescent Cell Viability Assay (Promega). All cell culture experiments were repeated three times unless otherwise noted. To inhibit MEK signaling, cells were treated with trametinib (ChemScene) at 1 or 10 nM in the medium. For the soft agar colony formation assay, 1–2 × 10 3 cells were mixed in 0.4% agar, seeded into 6-well plates, and cultured for 14 days. The cells were stained with Giemsa Stain Solution (Wako), and the numbers of colonies were counted under a dissecting microscope. Flow cytometry analyses The trypsin-dissociated single cells were prepared from organoids and fixed with 4% paraformaldehyde for 10 min. After being permeabilized in cold methanol, the cells were stained with Alexa Fluor 488-conjugated anti-cleaved caspase 3 antibody (Cell Signaling Technology) at 1:50 at room temperature for one hour. After washing, apoptotic cells were analyzed using a FACSCanto II (Becton Dickinson). DNA sequencing Genomic DNA was extracted from organoid cells. The genomic DNA fragment encompassing exons 7 and 8 of Trp53 was amplified by PCR using a primer set (p53F2 and p53R2). The DNA sequences around codon 270 of Trp53 was examined by direct sequencing using the forward primer. Genomic DNA from CMT93 cells (ATCC) was used as the Trp53 wild-type control. CGH analyses Genomic DNA was extracted and purified from the AKTP +/M and AKTP M/LOH cells, and the whole-genome CGH array was performed by a SurePrint G3 Mouse Genome CGH microarray 1 × 1 M (Agilent). Genotyping Trp53 in cell lines Genotyping of Trp53 in organoid cell lines was performed using a TaqMan SNP genotyping assay (Applied Biosystems). The custom TaqMan probes for wild-type Trp53 (VIC dye) and mutant Trp53 R270H (FAM dye) were designed in exon 8, including R270 codon of mouse Trp53 . The sequences of TaqMan probe and primers (p53F3 and p53R3) are provided below. The PCR results were analyzed by an allele discrimination/SNP analysis system in Mx3000P (Stratagene). Primer sequences used in the study: p53F1, agcctgcctagcttcctcagg ; p53R1, cttggagacatagccacactg ; p53F2, agactccaggtaggaaggcgcgtggta ; p53R2, cttggtcccgcctgcgtacctctcttt ; p53F3, ccggatagtgggaaccttctg ; p53R3, tcttctgtacggcggtctct . TaqMan probe used for Trp53 genotyping TaqMan MGB probe to detect wild-type Trp53 (VIC dye): CTTTGAGGTTC G TGTTTGT TaqMan MGB probe to detect mutant Trp53 R270H (FAM dye): CTTTGAGGTTC A TGTTTGT RNA sequencing and analyses Total RNA was extracted from organoid cells of AKTP M/LOH , and AKTP Null using an RNeasy plus Micro Kit (Qiagen). RNASeq libraries were prepared using a SureSelect Strand Specific RNA Reagent Kit (Agilent Technologies) according to the manufacturer’s protocol. Single-end sequencing with 50 cycles, such that adapters at 3’-ends of reads were not included, was performed using an Illumina HiSeq3000 (Illumina). All reads were demultiplexed on the basis of their unique indices using Illumina’s bcl2fastq2 (version 2.20). Sequencing data were deposited in the DNA Data Bank of Japan (DDBJ; accession #DRA005647 and #DRA008701). The quality of raw reads was assessed with FastQC (version 0.11.9) [38] ; the quality scores were >Q30, which indicated high quality (Supplementary Fig. 9a ). In data processing step, read deduplication was skipped because computational removal of read duplicates, especially in low quantity samples can worsen the power for the differential gene expression [39] , [40] . Clean reads, for which the average quality scores for A, AKTP +/+ , AKTP +/M , AKTP M/LOH and AKTP Null samples were greater than Q30, were processed using the Tuxedo protocol [41] with TopHat2 (version 2.1.1) [42] and Cufflinks [43] . To maintain the previous gene expression data of the A, AKTP +/+ , and AKTP +/M samples [26] with the splice junction rate in read alignment, reads for each sample were aligned to the mouse reference GRCm38.p4/mm10 using TopHat2 with the following arguments: (1) segment-length 17, (2) segment-mismatches 1 and (3) library-type fr-unstranded. Although the segment-length was adjusted (25 to 17), the mapping rate of AKTP M/LOH and AKTP Null reads with the two values was found to be almost similar (Supplementary Fig. 10 ). After sequence alignment, the duplication rate of reads was determined by sequence- and mapping-based approaches using RSeQC [44] , and the low distribution of uniquely mapped reads from mapping-based QC (11–18%) were observed (Supplementary Fig. 9b ), indicating high rates of read duplicates, possibly due to RNA-Seq library preparation with low input amounts. 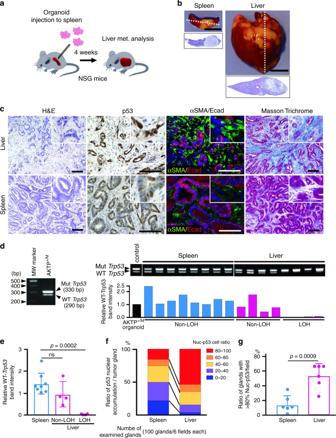Fig. 1: Enrichment ofTrp53LOH cells in liver metastasized tumor cells. aStrategy for liver metastasis development in NSG mice.bRepresentative photographs of the spleen and liver at 4 weeks after transplantation, and histology sections of dashed lines (H&E). Bars, 10 mm.cRepresentative histology of liver metastases (top) and primary spleen tumors (bottom). H&E, immunohistochemistry for p53, double-fluorescence immunostaining for α-smooth muscle actin (αSMA) and E-cadherin (Ecad) and Masson Trichrome staining (left to right). The insets show enlarged images. Bars, 100 µm.dRepresentative results of genomic polymerase chain reaction (PCR) forTrp53in AKTP+/Mcells (left) and spleen and liver tumors (right top). Each lane indicates the tumor cells collected from independent tumors in the spleen and liver. MutTrp53and WTTrp53indicate mutantTrp53R270H and wild-typeTrp53, respectively. The AKTP+/Morganoid DNA was used as control. The band intensities (WTTrp53/MutTrp53) were quantified using ImageJ, and relative band intensities of each sample in spleen (blue bars) and liver (magenta bars) to that of control (closed bar) are indicated as bar graph (n= 1 for each bar corresponding to each band) (bottom). LOH, loss of heterozygosity.eThe mean relative band intensities in spleen tumors (blue) and liver tumors (magenta) indicated in (d) are shown. Note that the level of the mean band intensity was significantly decreased in LOH tumors in the liver.fThe ratio of tumor cells with p53 nuclear-only accumulation in the spleen and liver tumors are indicated by different colors, blue, 0–20%; purple, 20–40%: yellow, 40–60%, orange, 60–80%, and red, 80–100%. The nuclear accumulation of p53 was examined in 100 tumor glands (>20 cells/gland) for 6 microscopic fields.gThe mean ratios of tumor glands containing nuclear-only p53 cells at >80% in spleen tumors (blue) and liver tumors (magenta) are shown. The data ine,gare presented as mean ± s.d. Two-sided unpairedt-test was used for statistical analysis.pvalues are provided; ns, not significant. Ine,n= 8 (spleen tumors) andn= 4 (non-LOH or LOH liver tumors) biologically independent samples. Ing,n= 6 biologically independent samples. Source data are provided as aSource datafile. The sequencing data are summarized in Supplementary Table 1 . Gene expression quantification was performed using Cufflinks [43] , and Reads Per Kilobase of transcript per Million mapped reads (RPKM) was calculated as the expression value. A principal component analysis (PCA) was performed on the basis of RPKM values to examine whether the samples clustered per their genotype differences (Supplementary Fig. 9c ). Differential expression analyses between samples with replicates were performed using Cuffdiff, with the cut-off set at P < 0.01 and ≥1.5-fold change (DEGs are presented in Supplementary Data 1 ), shown in the volcano plot of DEGs with statistical significance (Supplementary Fig. 9d ). Hierarchical clustering in the gene expression data was analyzed with MeV ( http://mev.tm4.org ) using Euclidean distance and the complete linkage method. For the upstream regulator analysis, the AKTP M/LOH - and/or AKTP Null -specific gene set was analyzed using the Ingenuity Pathway Analysis software package (Ingenuity Systems; www.ingenuity.com ). Pathways with z-scores of >2 (for inflammatory pathways) or >3 (for growth factor/MAPK pathways) and P -values of <0.05 were designated as significantly activated. Mutual exclusivity analysis Mutual exclusivity of TP53 mutation and FBXW7 mutation in the human colorectal cancer TCGA database was examined using cBioPortal ( https://www.cbioportal.org ). StemChecker analysis The stemness signature in AKTP +/M , AKTP Null and AKTP M/LOH was analyzed using StemChecker [45] , a web-based online tool for examining the stemness signatures in user-defined gene sets based on the curation of 50 published stemness signatures ( http://stemchecker.sysbiolab.eu ). STRING database analysis Genes that were predicted to be targeted by 31 upstream regulators (Fig. 7c, d ) were selected. For protein-protein interaction network analysis, those genes were searched against STRING database [46] with medium confidence score (>0.4). A pattern arising as a result of interactions between genes was visualized with a heatmap. Statistical analyses The data were analyzed using a two-sided unpaired t -test otherwise mentioned and presented as the means ± standard deviation (s.d.). 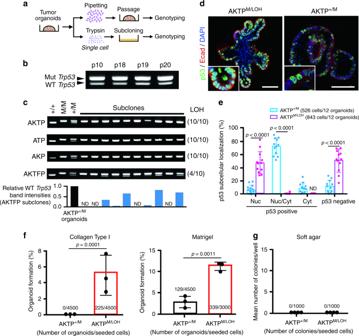Fig. 2: Selection ofTrp53LOH cells in the subcloned intestinal tumor cells. aSchematic drawing of theTrp53LOH analysis. The organoids were mechanically dissociated by pipetting and passaged into Matrigel or were enzymatically dissociated to single cells and subcloned on culture dishes.bRepresentative genomic PCR results ofTrp53of AKTP+/Morganoids maintained in Matrigel with mechanical passage (p, passage number). MutTrp53and WTTrp53indicate mutantTrp53R270H and wild-typeTrp53, respectively. Molecular weight marker forTrp53allele-specific PCR is shown in Fig.1d. The experiments shown in (b) were repeated three times with similar results, and the representative results are shown.cGenomic PCR results ofTrp53of independent subclones from AKTP+/M, ATP+/M, AKP+/M, and AKTFP+/Morganoids. Genomic DNAs of AKTP+/+, AKTPM/M, and AKTP+/Mcells were used as controls. The numbers ofTrp53LOH subclones per total subclones are indicated in parentheses. The band intensities (WTTrp53/MutTrp53) of AKTPF subclones were quantified using ImageJ, and relative band intensities of each subclone (blue bars) to that of control (closed bar) are indicated as bar graph (n= 1 for each bar corresponding to each band) (bottom). ND, not detected.dRepresentative confocal images of AKTPM/LOH(left) and AKTP+/M(right) organoids immunostained for p53 and E-cadherin (Ecad) with DAPI nuclear staining are shown. The insets indicate enlarged images. Bars, 100 µm.eThe percentages of p53 subcellular localization with nuclear-only (Nuc), mixed nuclear and cytoplasmic (Nuc/Cyt), and cytoplasmic-only (Cyt) in the AKTP+/M(blue) and AKTPM/LOH(magenta) organoid cells are shown. The total numbers of examined cells/organoids are indicated.fThe ratios of organoid development from single AKTP+/Mcells (closed bar) and AKTPM/LOHcells (red bars) in type I collagen gel (left) and Matrigel (right) are shown. The numbers of developed organoids and seeded cells are provided.gThe results of soft agar colony formation assay. The number of colonies and seeded cells are provided. The data ine,fare presented as mean ± s.d.,n= 12 (e) andn= 3 (f) biologically independent samples.pvalues are provided; ND, not detected. Two-sided unpairedt-test was used to calculate statistical difference. Source data are provided as aSource datafile. 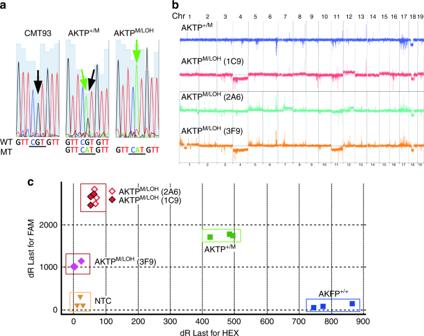Fig. 3: Mechanism underlyingTrp53LOH in AKTP+/Mcells. aDirect sequencing of genomic DNA fragments including codon 270 (under line) ofTrp53in CMT93 cells, AKTP+/M, and AKTPM/LOHcells. WT, wild-typeTrp53; and MT, mutantTrp53(R270H).bA whole-genome CGH analysis of the indicated AKTPM/LOHsubclones (1C9, 2A6, and 3F9) and parental AKTP+/Mcells. Chr indicates chromosome number.cTaqMan SNP genotyping results of AKTPM/LOH2A6 cells (open diamonds with red line), AKTPM/LOH1C9 cells (red diamonds with black line), AKTPM/LOH3F9 cells (magenta diamonds), AKTP+/Mcells (green squares), AKTP+/+cells (blue squares), and no template control (NTC) (yellow triangles) are shown as a scatter plot. TheTrp53allelic discrimination data are shown as a scatter plot ofTrp53wild-type codon 270 (CGT) (HEX dye) versusTrp53mutant codon R270H (CAT) (FAM dye). Note that two AKTPM/LOHsubclones (2A6 and 1C9) carry two copies of mutantTrp53R270H, while one AKTPM/LOHsubclone 3F9 carries one copy orTrp53R270H. Source data are provided as aSource datafile. Statistical analyses for Figs. 4 d, e and 7f were performed using a one-way ANOVA, followed by Tukey’s post-hoc test. Statistical analyses for Fig. 6c were performed using Wilcoxon’s nonparametric analysis. A value of p < 0.05 was considered to be statistically significant. 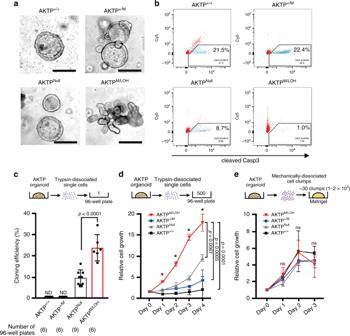Fig. 4: Increased survival of dissociated tumor cells byTrp53GOF mutation with LOH. aRepresentative photographs of four AKTP organoid lines with differentTrp53genotypes (AKTP+/+, AKTP+/M, AKTPNull, and AKTPM/LOH). Bars, 500 µm. Note that AKTPM/LOHcells formed a complex glandular structure, while other organoids showed a round cystic structure. The images are representative of six independent cultures.bA flow cytometry analysis for cleaved caspase 3 (Casp3) of trypsin-dissociated cells of the four differentTrp53genotypes. Gating strategy is shown in Supplementary Fig.5. The apoptosis rate is indicated in each graph.cCloning efficiencies examined by limiting dilution of trypsin-dissociated single cells in 96-well plates are shown as a bar graph. The numbers of 96-well plates used for each genotype analysis are indicated in parentheses. Cloning efficiency was calculated in each 96-well plate, and the mean cloning efficiency was calculated (n= 6–9 biologically independent samples). Gray-line bar, AKTPNullcells; red-line bar, AKTPM/LOHcells; and ND, not detected.d,eThe results of a cell proliferation assay of trypsin-dissociated single AKTP cells (500 cells/well) (n= 3 biologically independent samples) (d) and mechanically dissociated AKTP cell clumps (~30 clumps containing 1–2 × 103cells/Matrigel) (n= 3 biologically independent samples) (e). Red lines with triangles, AKTPM/LOHcells; blue lines with circles, AKTP+/Mcells; gray lines with triangles, AKTPNullcells; and black lines with squares, AKTP+/+cells. The relative cell growth compared to the day 0 level is indicated. Data are presented as mean ± s.d. The data incwere analyzed by two-sided unpairedt-test,pvalues are provided; ND, not detected. The data ind,ewere analyzed by ANOVA test, *p< 0.0001; ns, not significant. Data indwere also analyzed by Tukey test,pvalues at day 4 are provided. Source data are provided as aSource datafile. Excel (16.23, Microsoft) and Graphpad Prism7 were used for statistical analyses. 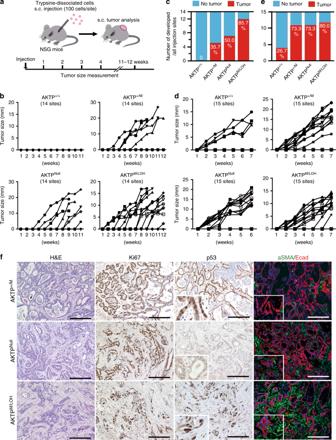Fig. 5: Enhanced tumor-initiating ability byTrp53GOF mutation with LOH. aStrategy of subcutaneous (s.c.) tumor development in NSG mice.bThe s.c. tumor size changes in each site injected with 1 × 102trypsin-dissociated cells of the indicated genotypes are shown as line graphs. The total number of injected sites (n= 14) is indicated in each graph. Each line with closed or open circles, squares, diamonds, or triangles indicates the kinetic tumor size development of an individual tumor.cThe total number of developed tumors (y-axis) at the 14 injected sites is shown by red bars. Blue bars indicate number of sites where tumors did not develop. The ratio (%) of tumor development is indicated inside each bar.dThe s.c. tumor size changes in each site injected with 5 × 103mechanically dissociated cells of the indicated genotypes are shown as line graphs. The total number of injected sites (n= 15) is indicated in each graph. Each line with closed or open circles, squares, diamonds, or triangles indicates the kinetic tumor size development of an individual tumor.eThe total number of developed tumors (y-axis) at the 15 injected sites is shown. The ratio (%) is indicated inside each bar.fRepresentative histology photographs of s.c. tumors that developed from 1 × 102trypsin-dissociated cells. Cell genotypes are indicated in the left. H&E and immunohistochemistry for Ki67, p53, and double fluorescent immunohistochemistry for α-smooth muscle active (αSMA) (green)/E-cadherin (Ecad) (red) are shown. The insets show enlarged images. Bars, 200 µm. Source data are provided as aSource datafile. 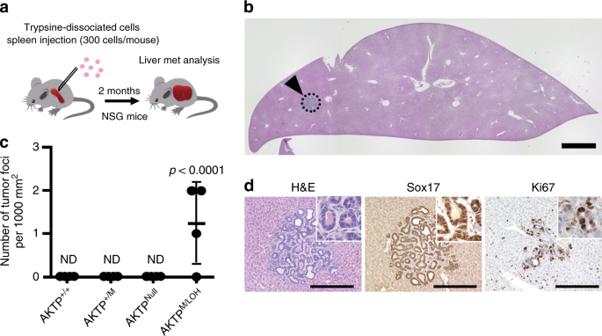Fig. 6: Enhanced metastasis-initiating ability of theTrp53GOF/LOH tumor cells. aThe strategy of metastasis tumor development in NSG mouse liver. A small number of trypsin-dissociated cells (3 × 102cells) were injected into the spleen. The liver metastatic foci were examined by an intensive histological analysis.bRepresentative histology section of the whole liver lobe of a mouse injected with AKTPM/LOHcells (H&E) is shown. The arrowhead indicates a micrometastatic lesion consisting of AKTPM/LOHcells. Bar, 1 mm. The image is a representative of three independent mice that showed liver metastasis.cThe numbers of metastatic tumor foci found in the liver in each mouse are shown with closed dots. Data are presented as mean ± s.d.,n= 4 biologically independent animals. Wilcoxon’s nonparametric analysis was used to calculate statistical difference.pvalue vs. AKTP+/+, AKTP+/M, and AKTPNullcells is provided; ND, not detected.dRepresentative histology of the serial sections of an AKTPM/LOHcell metastatic lesion (indicated lesion by dotted circle inb); H&E and immunohistochemistry for Sox17 and Ki67 (left to right). Bars, 200 µm. The images are representative of three independent experiments. Source data are provided as aSource datafile. 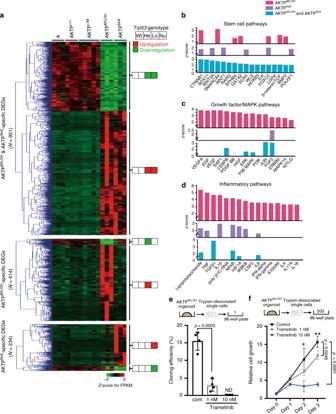Fig. 7: Activation of inflammatory and MAPK pathways byTrp53GOF mutation with LOH. aA hierarchical clustering analysis of AKTPM/LOHand AKTPNull-specific DEGs (top), AKTPM/LOH-specific DEGs (middle) and AKTPNull-specific DEGs (bottom) are shown as fold changes of RPKM compared with the mean. Color scale represents the Z-score log2 intensity. ForTrp53genotypes, Wt, AKTP+/+; He, AKTP+/M; Lo, AKTPM/LOH; and Nu, AKTPNull. The color in the squares on the right of heatmap indicates genes that are upregulated (red) or downregulated (green) compared to A organoid.b–dThe results of upstream regulator analyses by the Ingenuity Pathway Analysis software program using the AKTPM/LOH-specific DEGs (magenta bars), AKTPNull-specific DEGs (purple bars), and AKTPM/LOH& AKTPNull-specific DEGs (blue bars) mentioned in (a) are shown in bar graphs. Upstream regulators for the stem cell pathways with Z-scores > 2.0 in AKTPM/LOH& AKTPNull-specific DEGs (b), the growth factor/MAPK pathway with Z-scores > 2.0 (c) and the inflammatory pathway with Z scores > 3.0 in AKTPM/LOH-specific DEGs (d) are extracted and pathways with Z-scores > 1.5 are indicated as bars.eCloning efficiencies of trypsin-dissociated AKTPM/LOHcells in the presence or absence of trametinib examined by limiting dilution in 96-well plates are shown (n= 4 biologically independent samples).fThe results of a cell proliferation assay of trypsin-dissociated single AKTPM/LOHcells (500 cells/well) in the presence or absence of trametinib (mean ± s.d.) (n= 4 biologically independent samples). Data are presented as mean ± s.d. The data inewere analyzed by two-sided unpairedt-test,pvalue is provided; ND, not detected. The data infwere analyzed by ANOVA test, *p= 0.0994 at day 2, and **p= 0.0012 at day 3. The data infwere also analyzed by Tukey test,pvalues at day 3 are provided. Source data are provided as aSource datafile. 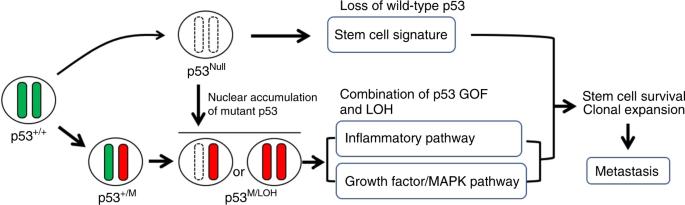Fig. 8: A schematic illustration of the forTP53/Trp53mutation and metastasis. Loss of wild-type p53 increases stemness, while combination of p53 GOF mutation with LOH activates inflammatory and MAPK pathway. Corporation of these pathways may cause acquisition of single-cell survival and clonal expansion abilities, which promotes metastasis. Reporting summary Further information on research design is available in the Nature Research Reporting Summary linked to this article.